RETRACTED ARTICLE: Selective inheritance of target genes from only one parent of sexually reproduced F1 progeny inArabidopsis Sexual reproduction constrains progeny to inherit allelic genes from both parents. Selective acquisition of target genes from only one parent in the F1 generation of plants has many potential applications including the elimination of undesired alleles and acceleration of trait stacking. CRISPR/Cas9-based gene drives can generate biased transmission of a preferred allele and convert heterozygotes to homozygotes in insects and mice, but similar strategies have not been implementable in plants because of a lack of efficient homology-directed repair (HDR). Here, we place a gene drive, which consists of cassettes that produce Cas9, guide RNAs (gRNA), and fluorescent markers, into the CRYPTOCHROME 1 ( CRY1) gene through CRISPR/Cas9-mediated HDR, resulting in cry1 drive lines. After crossing the cry1 drive /cry1 drive lines to wild type, we observe F1 plants which have DNA at the CRY1 locus from only the cry1 drive /cry1 drive parent. Moreover, a non-autonomous trans-acting gene drive, in which the gene drive unit and the target gene are located on different chromosomes, converts a heterozygous mutation in the target gene to homozygous. Our results demonstrate that homozygous F1 plants can be obtained through zygotic conversion using a CRISPR/Cas9-based gene drive. Sexually reproduced progeny acquire allelic genes from both parents. Sexual reproduction thus produces genetic variation and diversity among offspring. However, the heterozygosity in all loci of the sexually reproduced progeny poses a major challenge in crop breeding because traits segregate in subsequent generations according to Mendelian genetics, making it laborious and time consuming to fix and stack multiple traits. Developing technologies that enable selective inheritance of target genes from only one parent in the first generation will accelerate crop breeding. Such technologies can use fewer generations to fix traits and avoid certain detrimental alleles. CRISPR/Cas9-based gene drives can convert a heterozygote into a homozygote in Drosophila by zygotic conversion [1] and enable super-Mendelian inheritance of a target gene in both mice and insects by generating a bias of preferred gametes [1] , [2] , [3] , [4] , [5] . Therefore, gene drives can potentially be used to force selective acquisition of target genes from only one parent in plants through zygotic conversion. Canonical CRISPR/Cas9-based gene drives (sometimes called full drives or self-limiting drives) rely on the nuclease activities of Cas9 to generate a double-strand DNA break (DSB) in the target gene in one of the homologous chromosomes and use cellular DNA repair machinery to fix the DSB by copying the sequences from the other homologous chromosome [1] . The essence of CRISPR/Cas9-based gene drives is efficient Homology-Directed Repair (HDR) of DSBs [1] . It has been very difficult to conduct HDR in plants because Non-Homologous End Joining (NHEJ) is the predominant pathway for repairing DSBs [6] , [7] . However, recent findings indicate that the timing of DSB generation and the amount of Cas9 available are key determinants of HDR efficiency in Arabidopsis [8] , [9] . One strategy to increase cellular Cas9 concentrations is to transform an HDR construct into Arabidopsis lines that have already expressed Cas9 [8] . The timing of DSB generation can be controlled by using specific promoters to drive Cas9 expression. The DISRUPTION OF MEIOTIC CONTROL 1 ( DMC1 ) promoter [10] and the DD45/EC1.2 egg cell-specific promoter [11] , [12] are active during meiosis and early embryogenesis, respectively. Therefore, Cas9 expression under the control of the promoters may facilitate DSB generation at a particular developmental stage. Indeed, Cas9 expression driven by the DD45 promoter was previously demonstrated to increase HDR efficiency [8] , [13] . In this work, we design CRISPR/Cas9-based gene drives to test whether such gene drives can perform cutting and copying of genetic elements in Arabidopsis (Fig. 1a , Supplementary Figs. 1 and 2 ), and whether zygotic conversion can be achieved. We place the gene drive element, which produces Cas9, guide RNAs, and fluorescence markers, into the CRYPTOCHROME 1 ( CRY1 ) gene in Arabidopsis . We unequivocally show that up to 8% of the F1 plants, which are generated by crossing the homozygous gene drive line to WT, only have DNA from the gene drive line at the CRY1 locus, whereas all other loci in the genome contain an equal amount of DNA from each parent. Our results demonstrate that both copies of the target gene can come from a single parent while maintaining heterozygosity in all other loci. We further show that a trans-acting gene drive, which is placed in a location that is not linked to the target gene, also enables the F1 plants to inherit the target gene from only one parent. Fig. 1: A CRISPR/Cas9-based gene drive in Arabidopsis converts heterozygous plants into homozygous plants. a A schematic representation of the gene drive that is inserted into the second exon of the CRYPTOCHROME 1 ( CRY1 ) gene on Chromosome IV using CRISPR/Cas9-mediated homology-directed repair (HDR). The gene drive element flanked with homology arms is released by the Cas9/gRNA2 complex, which is produced by the Cas9 and gRNA units on the gene drive. The gene drive element has several components: a Cas9 -expressing unit, two gRNA units (one targeted CRY1 and the other was used to release the HDR template from the plasmid). The GFP gene is designed to fuse with part of CRY1 in frame, providing a visual marker for precise insertion of the gene drive element. The mCherry is another marker for selecting transgenic events. The Cas9 target sequence in CRY1 with the CCC (underlined) protospacer adjacent motif (PAM) is shown. The HDR events can be identified using PCR-based methods. Both P1 (CRY1-LA-GT-5P) and P4 (CRY1-RA-GT-3P) were located outside of the homology arms. b Conversion of heterozygous F1 plants into homozygous plants by the gene drive. The gene drive unit shown in a is shown in red here. When the homozygous gene drive line (♀), which was generated in the Columbia (Col) background (in black), was crossed to Landsberg (Ler, in blue), the F1 plants should contain just one copy of the gene drive at the CRY1 locus. When the gene drive functions as designed, the Cas9/gRNA complex cuts CRY1 in the Ler chromosome, and the gene drive element in the Col chromosome is copied into the Ler CRY1 locus, resulting in homozygous F1 plants. Full size image Large DNA fragments are precisely inserted into the genome via HDR The first step of constructing a gene drive line in Arabidopsis was to precisely place the gene drive constructs in a target gene. This experiment would also reveal whether we can achieve efficient HDR in Arabidopsis , a prerequisite for a functional gene drive. Our gene drive design consists of a Cas9 expression unit, two guide RNA (gRNA) units, and two fluorescent markers for selecting transgenic events and in-frame insertions (Fig. 1a , Supplementary Figs. 1 and 2 ). We previously showed that mCherry is a very effective marker for selecting transgenic Arabidopsis T1 seeds [14] . The gene drive element was flanked by an ~550 bp homology arm on each side (Fig. 1a , Supplementary Figs. 1 and 2 ). Two gRNAs were produced from the gene drive construct under the control of the Arabidopsis U6-26 and U6-29 promoters, respectively (Supplementary Figs. 1 and 2 ). The first gRNA targeted the second exon of the CRYPTOCHROME 1 ( CRY1 ) gene on Chromosome IV and the second gRNA was used to release the gene drive elements along with the homology arms (Fig. 1a ). We chose the CRY1 gene, which encodes a blue light photoreceptor, as our target gene because homozygous cry1 mutants have long hypocotyls when grown in light [15] , providing a visible phenotype for assessing genetic modifications at the CRY1 locus. We made two versions of the gene drive construct, which differed in the promoter used for driving Cas9 expression. Cas9 was under the control of the DMC1 promoter in one construct, and the other construct expressed Cas9 using the Egg-Cell ( EC ) specific promoter, which consisted of the EC1.2 enhancer and the EC1.1 promoter (Supplementary Figs. 1 and 2 ) [16] . 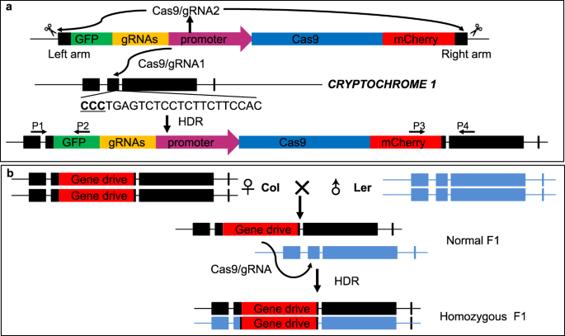Fig. 1: A CRISPR/Cas9-based gene drive inArabidopsisconverts heterozygous plants into homozygous plants. aA schematic representation of the gene drive that is inserted into the second exon of theCRYPTOCHROME 1(CRY1) gene on Chromosome IV using CRISPR/Cas9-mediated homology-directed repair (HDR). The gene drive element flanked with homology arms is released by the Cas9/gRNA2 complex, which is produced by the Cas9 and gRNA units on the gene drive. The gene drive element has several components: aCas9-expressing unit, two gRNA units (one targetedCRY1and the other was used to release the HDR template from the plasmid). TheGFPgene is designed to fuse with part ofCRY1in frame, providing a visual marker for precise insertion of the gene drive element. The mCherry is another marker for selecting transgenic events. The Cas9 target sequence inCRY1with the CCC (underlined) protospacer adjacent motif (PAM) is shown. The HDR events can be identified using PCR-based methods. Both P1 (CRY1-LA-GT-5P) and P4 (CRY1-RA-GT-3P) were located outside of the homology arms.bConversion of heterozygous F1 plants into homozygous plants by the gene drive. The gene drive unit shown inais shown in red here. When the homozygous gene drive line (♀), which was generated in the Columbia (Col) background (in black), was crossed to Landsberg (Ler, in blue), the F1 plants should contain just one copy of the gene drive at theCRY1locus. When the gene drive functions as designed, the Cas9/gRNA complex cutsCRY1in the Ler chromosome, and the gene drive element in the Col chromosome is copied into the LerCRY1locus, resulting in homozygous F1 plants. The two constructs were each transformed into two Cas9 -expressing lines, generating four combinations (Table 1 ). Table 1 Identification of an efficient strategy for HDR in Arabidopsis . Full size table We used PCR-based methods to identify T1 plants that had undergone HDR at the CRY1 locus (Supplementary Fig. 3 ). As shown in Table 1 , we observed HDR events in all four combinations with efficiencies ranging from 9.8% to 21.7%. However, the majority of the HDR events only occurred at one side of the homology arm (Table 1 ). When Cas9 in both the gene drive construct and in the background was driven by an egg cell-specific promoter ( EC or DD45 ), the highest efficiency was achieved (Table 1 ). We observed that 4.68% of the T1 transformants had the gene drive element precisely placed in the CRY1 gene via HDR (Table 1 ). The results further suggest that the DMC1 promoter is not as effective as the EC promoters. When only the DMC1 promoter was used to drive Cas9 expression in both the gene drive construct and in the background, we did not obtain any plants that had the gene drive construct precisely inserted inside the CRY1 gene (Table 1 ). To determine whether the entire gene drive unit, which was about 10 kb for the EC-Cas9 construct (Supplementary Fig. 1 ), was inserted into CRY1 , we used two long PCR reactions to amplify two overlapping fragments from the line EC-Cas9/DMC1 #128 ( EC-Cas9 refers to the Cas9 unit in the gene drive construct and DMC1 represents the DMC1-Cas9 unit in the Arabidopsis background) (Fig. 1a , Supplementary Fig. 4 ). Two of the primers were located outside of the homology arms so that the gene drive element in the original plasmid would not be amplified (Fig. 1a , Supplementary Fig. 4 ). Sequencing of the fragments confirmed that the intended gene drive was precisely inserted into the CRY1 gene through HDR. These results demonstrated that it is feasible to target large DNA fragments to a desired locus in Arabidopsis , providing useful tools for plant engineering and synthetic biology. The EC-Cas9/DMC1 #128 could thus be used to test whether our gene drive can function as designed in Arabidopsis . Full gene drives facilitate zygosity conversion We first selected a T2 plant of EC-Cas9/DMC1 #128 that was homozygous for the insertion of the gene drive element at the CRY1 locus (Fig. 1b ). We crossed the plant to the Landsberg (Ler) ecotype, which is polymorphic to the Columbia (Col) ecotype in which the EC-Cas9/DMC1 #128 line was generated. If our gene drive functioned as designed, we expected that the Cas9/gRNA complex would generate a DSB in the Ler CRY1 locus and the gene drive element would be used to repair the DSB through HDR, resulting in homozygous F1 plants at the CRY1 locus (Fig. 1b ). Note that the Cas9/gRNA complex does not target the DNA of the CRY1 locus once the gene drive element is inserted into CRY1 . Among the 195 F1 plants generated from pollination of the EC-Cas9/DMC1 #128 plant (♀) with Ler pollen, five were homozygous based on our PCR-based genotyping results. To distinguish the real F1 plants from those that resulted from self-pollination of EC-Cas9/DMC1 #128, we used DNA markers that differentiate Ler DNA from Col DNA. Results from using the marker T32M21, which is located on Chromosome V, demonstrated that the five homozygous plants were indeed F1 plants, which had both Ler and Col DNA at the T32M21 location (Supplementary Fig. 5 ). If the homozygous F1 plants resulted from using the Col allele as a template to repair the DSB in the Ler allele, we expected that only the gene drive element and its immediate neighboring sequence would be copied from the Col chromosome into the Ler chromosome and the rest of Chromosome IV should have Col DNA in one chromosome and Ler in the other homologous chromosome (Fig. 2a ). Results of analyzing the DNA markers upstream and downstream of the CRY1 locus indicated that both Col and Ler DNA were present in those locations, further demonstrating that Cas9/gRNA cut the Ler allele of CRY1 , and the DNA from the Col CRY1 locus was used as the template to repair the DSB through HDR (Fig. 2a ). Fig. 2: Determination of the molecular nature and sources of DNA in the homozygous F1 plants. a The homozygous F1 plants are truly generated by HDR in the F1 generation. The homozygous plants contain one copy of Ler DNA and one copy of Col DNA in all regions except for the CRY1 locus, where both copies of DNA were from the Col parent. The CIW5, F17A8, and F8B4 are Simple Sequence Length Polymorphism (SSLP) markers that can differentiate Col DNA from Ler DNA. The genotyping experiments were repeated three times. b Estimation of the break points of HDR by analyzing DNA markers located within the homology arms, which were used to place the gene drive element inside the CRY1 gene through HDR. The Cleaved Amplified Polymorphic Sequence (CAPS) marker LA uses the BslI enzyme to cut Ler DNA, but Col DNA is not digestible by BslI. The RA marker, which is 160 bp away from the gene drive element, can differentiate Col DNA from Ler when BamHI digestion is used. Genomic DNA was used as the PCR template. The PCR fragments were then digested with the corresponding enzymes. H refers to DNA from F1 plants generated from a cross between wild type Ler and wild type Col. The genotyping experiments were repeated three times. Source data are provided as a Source Data file. Full size image We identified two polymorphic regions in the homology arms that can be used as DNA markers (Fig. 2b , Supplementary Fig. 6 ) to differentiate Ler and Col DNA. The LA marker, which is located in the left homology arm and which is 140 bp from the gene drive element, revealed that all five F1 plants shown in Fig. 2a only had Col DNA at that location, clearly indicating that the region was copied from the Col chromosome. In contrast, three of the F1 plants at the RA marker contained both Col and Ler DNA (Fig. 2b ). The RA marker is located in the right homology arm and is 160 bp away from the gene drive element (Fig. 2b , Supplementary Fig. 6 ). Our results demonstrated that some F1 plants had only Col DNA at the marker locations while some F1 plants had both Ler and Col at the locations (Fig. 2 ). To further confirm the genotyping results, we sequenced the polymorphic regions of both the left and right arms (Supplementary Fig. 7 ). Consistent with the results of the LA and RA markers, the left arm of the 5 F1 plants only had Col DNA and three of the five F1 plants had both Ler/Col DNA in the right arm (Supplementary Fig. 7 ). To sequence the HDR junctions, we amplified a fragment that covered the entire left arm and part of the GFP gene (Supplementary Fig. 8 ). The Sanger sequencing results clearly showed that the gene drive element along with the left arm was perfectly copied into the Ler chromosome (Supplementary Fig. 8 ). We conducted similar experiments on the right side using a primer in the mCherry gene and a primer outside the right homology arm (Supplementary Fig. 8 ). The junctions at the right side appeared more complex than we expected. When we used the primer pair CRY1-MCR-RA5P/CRY1-RA-GT-3P (Supplementary Fig. 7 ), the resulting fragment contained both Col and Ler DNA for plants #24, #52 and #156 while only Col DNA for plants #15 and #30 (Supplementary Fig. 7 ). However, when the primer pair mCH-RA-GT-5P/CRY1-RA-GT-3P was used, the amplified DNA fragments in all F1 plants only contained Col DNA (Supplementary Fig. 8 ), suggesting that the three F1 plants, which contained Ler DNA in the right arm region, probably had imperfect HDR events. The exact nature of the HDR junction of the right side in the three F1 plants has not been resolved. Consistent with the results of T1 plants shown in Table 1 in which the majority of HDR events occurred only on one side, the copying mechanism mediated by the gene drive could also sometimes result in imperfect HDR. We noticed that there are multiple polymorphic regions in the right homology arm between Col/Ler (Supplementary Fig. 9 ). Moreover, there is a 3 bp deletion, which is located 74 bp away from the gene drive/right arm junction. It is well known that mismatches in homology arms can dramatically affect HDR efficiency [17] . The observed polymorphisms in the right arm might partially account for the observed imperfect HDR events in the three F1 plants. Gene editing in plants mediated by CRISPR/Cas9 often results in mosaic plants in the first generation [14] , [18] . To further confirm that the five F1 homozygous plants shown in Fig. 2 were not mosaic, we analyzed at least 48 F2 progeny resulting from self-pollination of each identified homozygous F1 plant. All of the light-grown F2 plants had the cry1 phenotype and were confirmed to be homozygous via PCR-based genotyping results, suggesting that the F1 parents were true homozygotes. Zygosity conversion efficiency depends on maternal Cas9 levels To test whether the gene drive element can be transmitted through the male side, we used pollen from the homozygous EC-Cas9/DMC1 #128 plant to perform crosses to wild type Ler. We genotyped 384 F1 plants and they were all heterozygous at the CRY1 locus, suggesting that the gene drive did not function efficiently through the male side. To test whether the gene drive can generate biased inheritance of a preferred allele, we analyzed the F2 population generated from self-pollination of a single heterozygous F1 plant of the EC-Cas9/DMC1 #128 (♀) x Ler (♂) cross (Fig. 3 ). We observed that 37.2% (123) of the 331 F2 plants tested were homozygous for the insertion at the CRY1 locus, which was significantly higher than the expected 25% Mendelian ratio ( p = 1.2 × 10 −6 , one-sample binomial test). Interestingly, the number of wild type plants ( CRY1/CRY1 ) in the F2 population was close to what is expected from Mendelian segregation (22.4% (74) vs 25% expected, p = 0.28, one-sample binomial test). Our results suggested that the observed additional homozygous cry1/cry1 plants were mainly generated by converting heterozygous ( CRY1/cry1 ) plants into homozygous plants by the gene drive (Fig. 3 ). This interpretation was consistent with the observation that only 40.4% of plants were heterozygous compared to the expected 50% ratio (Fig. 3 ). We further estimated NHEJ events in the population by taking advantage of the fact that loss-of-function cry1 mutants have long hypocotyls when grown in light. Plants with one copy of the gene drive insertion and one copy of CRY1 that had undergone NHEJ repair resulting in a frameshift ( cry1/cry1 *) displayed cry1 phenotypes. More than 35% of the F2 plants had loss-of-function NHEJ events, which occurred much more frequently than the observed HDR events (12.2%) (Fig. 3 ). Note that the apparent CRY1/CRY1 plants might also contain NHEJ events that did or did not result in a frameshift ( CRY1/cry1 ‡ and CRY1/cry1 *). The small number of ( cry1/cry1 ‡ ) might also contain NHEJ events such as three base pair deletions ( cry1/cry1 ‡ ) that did not result in loss of function. Therefore, the number of NHEJ events presented above was likely underestimated. Fig. 3: Biased inheritance mediated by a CRISPR/Cas9-based gene drive. A plant with a wild type (WT) CRY1 copy in one chromosome and the gene drive element (red) inserted in CRY1 in the homologous chromosome underwent self-pollination to produce progeny. Several genotypes are expected: both copies of CRY1 are WT ( CRY1/CRY1 ); one copy of CRY1 had NHEJ without disrupting CRY1 function such as a 3 bp deletion ( cry1 ‡ ); one copy of CRY1 had NHEJ resulting in loss of CRY1 function ( cry1 * ); heterozygous cry1 ; homozygous cry1 ; and plants with one copy of the gene drive insertion and one copy of cry1 that had undergone NHEJ repair ( cry1/cry1 *) that disrupted CRY1 function. The genotypes of CRY1/CRY1 , CRY1/cry1 ‡ , CRY1/cry1*, CRY1/cry1, and cry1/cry1 ‡ were not phenotypically different. Plants with either cry1/cry1 or cry1/cry1 * genotypes display long hypocotyls in light conditions. Full size image As discussed above, CRISPR/Cas9 edited plants are often mosaic in the first generation [14] , [18] . An alternative interpretation of the observed biased segregation among the F2 plants is that the F1 plants might be mosaic, which can also cause deviations from Mendelian ratios as we had previously observed in T2 plants [14] . It is difficult to resolve the two possibilities with experimental approaches. Our results suggest that the allelic conversion mainly took place in the early developmental stages of zygotes. The allelic conversion likely did not occur before or during meiosis because we observed the expected number of wild type plants. It appeared that if there was enough Cas9 and gRNA in the fertilized egg or initial developmental stages of the zygote, zygosity conversion could take place. To test this hypothesis, we crossed EC-Cas9/DMC1 #128 (♂) to the DD45-Cas9 line (♀), which already expresses Cas9 in egg cells. Among the 192 F1 plants analyzed, two had the homozygous insertion at the CRY1 locus. As discussed above, no homozygous F1 plants were identified when EC-Cas9/DMC1 #128 (♂) was crossed to Ler (♀), which does not have Cas9 in the egg cells. Our results suggest that the presence of Cas9 in the egg cell might facilitate successful early zygotic HDR in Arabidopsis . We also conducted similar analyses using the EC-Cas9/DD45 #83 line ( EC-Cas9 was in the gene drive construct) and the DMC1-Cas9/DD45 #189 line by crossing the homozygous T2 plants (♀) to Ler (♂). Our long PCR reactions similar to that shown in the Supplementary Fig. 4 confirmed that the complete gene drive elements were present in the two lines. 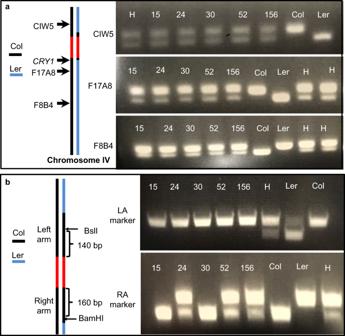Fig. 2: Determination of the molecular nature and sources of DNA in the homozygous F1 plants. aThe homozygous F1 plants are truly generated by HDR in the F1 generation. The homozygous plants contain one copy of Ler DNA and one copy of Col DNA in all regions except for theCRY1locus, where both copies of DNA were from the Col parent. The CIW5, F17A8, and F8B4 are Simple Sequence Length Polymorphism (SSLP) markers that can differentiate Col DNA from Ler DNA. The genotyping experiments were repeated three times.bEstimation of the break points of HDR by analyzing DNA markers located within the homology arms, which were used to place the gene drive element inside theCRY1gene through HDR. The Cleaved Amplified Polymorphic Sequence (CAPS) marker LA uses the BslI enzyme to cut Ler DNA, but Col DNA is not digestible by BslI. The RA marker, which is 160 bp away from the gene drive element, can differentiate Col DNA from Ler when BamHI digestion is used. Genomic DNA was used as the PCR template. The PCR fragments were then digested with the corresponding enzymes. H refers to DNA from F1 plants generated from a cross between wild type Ler and wild type Col. The genotyping experiments were repeated three times. Source data are provided as a Source Data file. For the EC-Cas9/DD45 #83 line, 8.13% of F1 plants were homozygous (Table 2 ). The cross between Ler (♂) and the DMC1-Cas9/DD45 #189 line (♀) resulted in 3.08% homozygous F1 plants (Table 2 ). Our DNA marker analyses demonstrated that the plants analyzed here were generated from the intended crosses and were F1 plants (Supplementary Fig. 10 ). Our results demonstrated that production of Cas9 from the egg cell-specific promoter increased efficiency in both gene targeting (Table 1 ) and zygosity conversion (Table 2 ). When both the gene drive construct and the Arabidopsis line for transformation used an egg cell-specific promoter to drive Cas9 expression, the highest efficiencies were observed (Tables 1 and 2 ). We further analyzed 262 plants that were generated by self-pollination of a single heterozygous F1 plant of the of DMC1-Cas9/DD45 #189 (♀) x Ler (♂) cross. We observed that 30.9% (81) of the F2 plants were homozygous for the gene drive element, indicating that biased segregation was also achieved ( p = 0.032, one-sample binomial test). Table 2 The effects of promoters used for Cas9 expression on the efficiencies of zygosity conversion. Full size table Non-autonomous trans-acting gene drives function in Arabidopsis Our analyses of the above gene drive lines demonstrated that a CRISPR/Cas9-based gene drive can be used to drive zygosity conversion and biased transmission of a preferred allele. However, a canonical gene drive and its target gene are located in the same locus, making them inseparable. We next designed a non-autonomous trans-acting gene drive that spatially separates the drive and target locus (Fig. 4a ). In a non-autonomous trans-acting gene drive, Cas9 and gRNA are arranged in tandem at the same location in the genome, but the drive acts on a target region different from where the drive is located (Fig. 4a ). The advantage of the non-autonomous trans-acting gene drive over the canonical gene drive is that the transgenes can be removed by genetic segregation once the target gene has been modified. Fig. 4: Non-autonomous trans-acting gene drives in Arabidopsis . a A schematic representation of a non-autonomous trans-acting gene drive. A Cas9 unit and a gRNA unit are placed in a location far away from the target gene (on a different chromosome). The Cas9/gRNA complex cuts the wild type allele of the target gene. Subsequently, the DSB is repaired using the DNA from the homologous chromosome as the template, resulting in a homozygous plant. b The NPY5-GFP line can be used to test a non-autonomous trans-acting gene drive in Arabidopsis . The line contains an EC-Cas9 unit and a gRNA unit on Chromosome II while the target wild type NPY5 is on Chromosome IV. The NPY5 gene has been tagged with GFP . The DD45-Cas9 unit on Chromosome V may provide additional Cas9 for the non-autonomous trans-acting gene drive. c The functionality of the non-autonomous trans-acting gene drive was tested by crossing the NPY5-GFP line to wild type Ler. Cas9/gRNA from Chromosome II cuts wild type NPY5 , generating a DSB. The GFP and DNA flanking GFP is used as a template for HDR, resulting in homozygous NPY5-GFP F1 plants. Full size image We previously used our HDR-based gene targeting technology to insert a GFP gene immediately before the stop codon of the NAKED PINS IN YUC MUTANTS 5 ( NPY5 ) gene, which is involved in auxin-mediated flower development [19] , [20] . We performed whole genome sequencing of the NPY5-GFP line and discovered that there were three transgene fragments in the genome (Fig. 4b , Supplementary Fig. 11 ). The GFP gene was precisely inserted in the NPY5 gene on Chromosome IV via HDR, as intended in our design (Fig. 4b , Supplementary Fig. 11 ). The second set of transgenes, which originated from the plasmid that was used to express Cas9 from the DD45 promoter [8] , was located at the end of Chromosome V (Fig. 4b , Supplementary Fig. 11 ). The third set of transgenes was inserted into Chromosome II and it came from the HDR construct for inserting the GFP gene in NPY5 (Fig. 4b , Supplementary Fig. 11 ). Further analysis of the transgene locus on Chromosome II revealed that the EC-Cas9 unit and the gRNA-producing unit targeting wild type NPY5 gene were still intact whereas the GFP and the homology arms had been excised (Supplementary Fig. 11 ). The NPY5-GFP line appeared ideal for us to test whether the Cas9 and gRNA units on Chromosome II could serve as a non-autonomous trans-acting gene drive to target NPY5 on Chromosome IV. We envisioned that Cas9 and gRNA, expressed from the locus on Chromosome II, would cut WT NPY5 and the DSB would be repaired using the template from the homologous chromosome (Fig. 4c ). We crossed the NPY5-GFP line (♀) to Ler (♂) and analyzed the zygosities of the F1 plants at the NPY5 locus. Among the 240 F1 plants analyzed, 9 were homozygous for NPY5-GFP . DNA marker analysis revealed that 3 of the homozygous plants were F1 plants resulting from the cross and that the rest of the plants were generated from self-pollination of the NPY5-GFP line (Supplementary Fig. 12 ). Our results demonstrated that a non-autonomous trans-acting gene drive can convert a heterozygous locus into a homozygous locus. We further sequenced the HDR junctions of the three homozygous F1 plants. They were all homozygous with precise HDR junctions (Supplementary Fig. 13 ), consistent with our PCR-based results (Fig. 4 ). We also genotyped the F2 progeny from the three homozygous plants and the F2 plants were all homozygous, consistent with an early HDR event or full zygotic conversion, rather than mosaicism. We clearly demonstrate that an existing allele of a target gene can be copied into the target gene of the homologous chromosome using CRISPR/Cas9-based gene drives (Figs. 1b and 4 ). 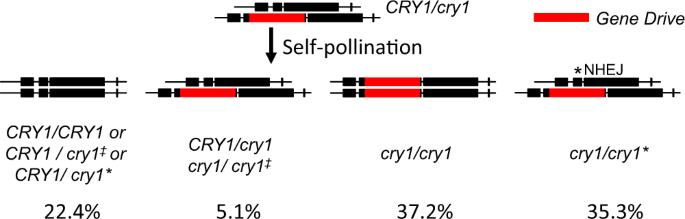Fig. 3: Biased inheritance mediated by a CRISPR/Cas9-based gene drive. A plant with a wild type (WT)CRY1copy in one chromosome and the gene drive element (red) inserted inCRY1in the homologous chromosome underwent self-pollination to produce progeny. Several genotypes are expected: both copies ofCRY1are WT (CRY1/CRY1); one copy ofCRY1had NHEJ without disruptingCRY1function such as a 3 bp deletion (cry1‡); one copy ofCRY1had NHEJ resulting in loss ofCRY1function (cry1*); heterozygouscry1; homozygouscry1; and plants with one copy of the gene drive insertion and one copy ofcry1that had undergone NHEJ repair (cry1/cry1*) that disruptedCRY1function. The genotypes ofCRY1/CRY1,CRY1/cry1‡, CRY1/cry1*, CRY1/cry1, and cry1/cry1‡were not phenotypically different. Plants with eithercry1/cry1orcry1/cry1* genotypes display long hypocotyls in light conditions. 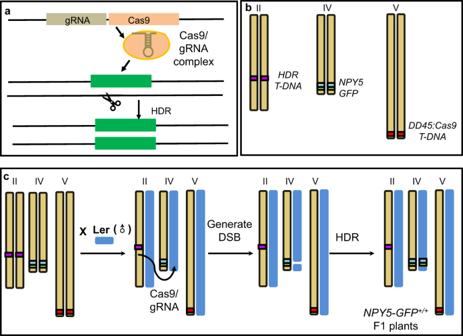Fig. 4: Non-autonomous trans-acting gene drives inArabidopsis. aA schematic representation of a non-autonomous trans-acting gene drive. ACas9unit and a gRNA unit are placed in a location far away from the target gene (on a different chromosome). The Cas9/gRNA complex cuts the wild type allele of the target gene. Subsequently, the DSB is repaired using the DNA from the homologous chromosome as the template, resulting in a homozygous plant.bTheNPY5-GFPline can be used to test a non-autonomous trans-acting gene drive inArabidopsis. The line contains anEC-Cas9unit and a gRNA unit on Chromosome II while the target wild typeNPY5is on Chromosome IV. TheNPY5gene has been tagged withGFP. TheDD45-Cas9unit on Chromosome V may provide additional Cas9 for the non-autonomous trans-acting gene drive.cThe functionality of the non-autonomous trans-acting gene drive was tested by crossing theNPY5-GFPline to wild type Ler. Cas9/gRNA from Chromosome II cuts wild typeNPY5, generating a DSB. TheGFPand DNA flankingGFPis used as a template for HDR, resulting in homozygousNPY5-GFPF1 plants. The copying of the preferred sequences can be achieved through either the canonical CRISPR/Cas9-based gene drives in which the Cas9 and gRNA units are inserted in the target gene (Fig. 1 ) or through non-autonomous trans-acting gene drives (Fig. 4a ). Our non-autonomous trans-acting gene drive makes it feasible to combine two existing alleles that are conferred by two tightly linked genes by copying one allele into the homologous chromosome in the F1 generation. Identification of additional promoters that can drive Cas9 expression at a time when HDR is favored over NHEJ will likely also help improve the efficiency of gene drives in plants. Plant materials and growth conditions The DD45-Cas9 transgenic line was obtained from Dr. Jian-kang Zhu and was previously described [8] . The DMC1-Cas9 transgenic line was generated by transforming Arabidopsis (Columbia ecotype) with a plasmid containing the DMC1-Cas9 unit. Both the DD45-Cas9 and DMC1-Cas9 lines were used for transformation of the gene drive constructs. Seeds were surface-sterilized and sown on vertical square plates with half-strength Murashige and Skoog (MS) medium (1/2 MS salts, 1.5% sucrose, 0.65% agar). They were stratified in the dark at 4 °C for 2 days, and then grown at 22 °C under a 16-h light/ 8-h dark cycle in a plant growth room. Plasmid construction An mCherry gene under the control of a seed-specific At2S3 promoter was cloned into the plasmid pHEE401E to generate pHEE401E-mCherry [14] , [16] . The two gRNA units, which produce one gRNA from the Arabidopsis U6-26 promoter and one gRNA from the U6-29 promoter, were cloned into the BsaI site in pHEE401E-mCherry by Gibson assembly. We then amplified the left homology arm of CRY1 , GFP , and the NOS terminator. We assembled the three fragments together by overlapping PCR reactions. The assembled fragment was then cloned into the HindIII site of the plasmid by Gibson assembly. Finally, the right homology arm of CRY1 was cloned into the EcoRI site of the plasmid that has the gRNA units and the left homology arm. The plasmid was called EC-Cas9 gene drive construct. The EC-Cas9 gene drive construct was digested with SpeI and XbaI to remove the EC promoter. The Arabidopsis DMC1 promoter was then cloned into the gene drive plasmid by Gibson assembly to generate the DMC1/Cas9 gene drive construct. For constructing the NPY5-GFP non-autonomous trans-acting gene drive lines, we used the backbone vector pHEE401E-mCherry [14] , [16] . We cloned two gRNA-producing units into the BsaI site (one gRNA targets NPY5 , the other gRNA was used to release the HDR template). We assembled the GFP gene flanked with two homology arms of NPY5 into the Hind III site. All of the primers used in this study are described in Supplementary Table 1 . Sequential plant transformation The gene drive constructs were transformed into Arabidopsis lines that have already harbored a Cas9 unit under the control of either the DD45 promoter or the DMC1 promoter. The strategy was previously described [8] . Transgenic T1 plants were selected using a second antibiotic/herbicide selection marker [8] . We screened the seeds harvested from plants that had undergone floral dipping using the mCherry fluorescent marker, as previously described [14] . Genotyping To identify T1 plants that contain the gene drive element in the CRY1 gene, we used PCR-based methods. We used the CRY1-LA-GT-5P/GFP-GT2 (CRY1-LA-GT-5P is located outside of the left homology arm) primer pair to amplify the left side HDR junction. We used the primer pair mCH-RA-GT-5P/CRY1-RA-GT-3P (CRY1-RA-GT-3P is outside of the right homology arm) to amplify the right HDR junction. To determine the zygosities of the gene drive plants, we used the CRY1-LA-GT-5P/CRY1-RA-GT-3P primer pair, which can amplify a fragment from both WT and heterozygous plants. To determine whether the entire gene drive element was inserted into CRY1 as designed, we amplified the entire insertion using two overlapping PCR reactions using the Q5 polymerase (Catalog, M0492S, NEB). One PCR product was amplified using the pHEE-CAS9-1361-5P/CRY1-RA-SEQ-3P primer pair (CRY1-RA-SEQ-3P is located outside of the right homology arm). The other side was amplified using CRY1-LA-SEQ-5P/ pHEE-CAS9-1474-3P primer pair. The two PCR products had a 113 bp overlap region. Testing gene drive functions via crosses The gene drive lines were crossed to Ler ecotype and the resulting F1 plants were genotyped using PCR-based methods. The primers were listed in Supplementary Table 1 . To confirm the genotypes and to eliminate the possibility of mosaicism in the identified homozygous F1, each homozygous plant was sampled three times at different growth stages. SSLP markers T32M21 (Chromosome V), CIW5, F17A8, AP22, T18I19, and F8B4 were used to differentiate Col and Ler DNA (Supplementary Table 1 ). To genotype the NPY5-GFP lines, the NPY5-GFP-MHGT1/NPY5-GFP-MHGT2 primers were used. Statistical analysis The two-sided one-sample binomial tests were performed by assuming Mendelian homozygous and wild type rates of 25% each after a heterozygous self-pollination. Stated p values represent the probability of observing proportions at least as extreme as those reported under the assumption that the proportions reflect Mendelian segregation. Values below 0.05 were deemed significant. Whole genome sequencing High molecular weight (HMW) DNA was extracted from four-week-old plants using a modified bomb protocol ( https://bomb.bio/protocols/ ). Two independent lines for NPY5-GFP and DD45-Cas9 were sequenced using both Oxford Nanopore Technologies (ONT; Oxford, UK) long read sequencing and Illumina (Illumina, Inc., San Diego, USA) short read sequencing. Unsheared HMW DNA was used to make barcoded ONT ligation-based libraries. Libraries were prepared starting with 1.5 µg of DNA and following all other steps in ONT’s SQK-LSK109 protocol. Final libraries were loaded on a ONT flowcell (v9.4.1) and run on the ONT PromethION sequencer (PromethION software (Minknow v19.12.5). Bases were called in real-time on the PromethION using the flip-flop version of Guppy (v3.1). The resulting fastq files were concatenated (fail and pass) and used for downstream genome assembly steps. Illumina short read libraries were prepared from sheared HMW DNA using NEBnext (NEB, Beverly, MA) and paired-end sequencing (2 × 150 bp) was generated on Illumina NovaSeq (Illumina, San Diego, CA). Genomes were assembled several different ways in order to identify all of the transgenes. Long read assemblies were carried out with Flye (v2.6) ( https://github.com/fenderglass/Flye ) and Miniasm (v0.3) ( https://github.com/lh3/miniasm ), while short reads were assembled with SPAdes (v 3.14.0) ( https://github.com/ablab/spades ), all using default settings. Flye long read assemblies were also polished using three rounds of racon with the input ONT reads (v1.4.13) and three rounds of pilon (v1.23) with the Illumina short reads. Transgene sequences were identified in the assemblies using BLAST (Blast+ v2.8.1) (ftp://ftp.ncbi.nlm.nih.gov/blast/executables/blast+/LATEST/) and adjacent sequences on the assembled contig were used to place the transgenes at specific genomic loci. Reporting summary Further information on research design is available in the Nature Research Reporting Summary linked to this article.